Enzymatic synthesis of benzylisoquinoline alkaloids using a parallel cascade strategy and tyrosinase variants Benzylisoquinoline alkaloid derived pharmaceuticals are widely applied in modern medicines. Recent studies on the microbial production of benzylisoquinolines have highlighted key biological syntheses towards these natural products. Routes to non-natural benzylisoquinolines have been less explored, particularly halogenated compounds which are more challenging. Here, we show the use of a tyrosinase, tyrosine decarboxylase, transaminase, and norcoclaurine synthase which are combined in a parallel cascade design, in order to generate halogenated benzylisoquinoline alkaloids in high enantiomeric excess. Notably, mutagenesis studies are applied to generate tyrosinase mutants, which enhance the acceptance of halogenated tyrosines for use in the biocatalytic cascades developed. Benzylisoquinoline alkaloids (BIAs) play an important role in the field of natural products due to their pharmaceutical properties. The use of plants containing BIAs dates back to 1500 BC, when the ancient Egyptians used opium as a painkiller [1] . Modern medicine revealed the biologically active components as codeine and morphine, both of which exhibit analgesic properties [2] , [3] . Recent studies on alkaloids have largely accelerated the use of BIA-derived pharmaceuticals, such as the anti-cancer agents noscapine and berberine [4] , [5] , anti-HIV agents coclaurine and norcoclaurine [6] , and anti-inflammatory drugs berbamine and coptisine [7] , [8] . Indeed, amongst all approved small-molecule based new drugs from 1981 to 2019, over 30% were based on natural products and 82% of these were semi-synthesised from natural product skeletons [9] Naturally-derived BIAs include around 2500 known compounds derived from the key intermediate ( S )-norcoclaurine, ( S )- 1 [10] . In plants, ( S )- 1 is produced by the condensation between dopamine 2 and 4-hydroxyphenylacetaldehyde (4-HPAA) 3 via a norcoclaurine synthase (NCS) mediated Pictet-Spengler reaction. Both 2 and 3 are derived from L-tyrosine 4 , via L-DOPA 5 and 4-hydroxyphenylpyruvic acid 6 by tyrosine hydroxylase (TH)/DOPA decarboxylase (DDC) and tyrosine aminotransferase (TyrAT)/4-hydroxyphenylpyruvate decarboxylase (4-HPPDC) respectively (Fig. 1a together with some examples of alkaloids formed) [11] , [12] . Fig. 1: Biosynthetic and biocatalytic routes to BIAs and a parallel cascade adopted in this work. a Biosynthetic BIA pathway in plants and examples of the alkaloid formed. L-Tyrosine 4 is converted to L-DOPA 5 by tyrosine hydroxylase (TH), then to dopamine 2 by DOPA decarboxylase (DDC). In a parallel pathway, 4 is converted into 4-HPAA 3 via 4-hydroxyphenylpyruvic acid 6 by tyrosine aminotransferase (TyrAT) and 4-hydroxyphenylpyruvate decarboxylase (4-HPPDC). Compounds 2 and 3 are condensed by the Pictet-Spenglerase norcoclaurine synthase (NCS), generating ( S )-norcoclaurine, ( S )- 1 , which is converted into BIAs, such as morphinans, aporphines and protoberberines [11] , [12] . b Cascade reactions to BIAs inspired by nature: i. Previous work on in vitro assembly of natural and non-natural BIAs from single amino acid substrate. ii. The in vitro parallel cascade to non-natural BIAs reported in this study. Full size image The reconstruction of heterologous BIA pathways into microbes is an exciting area of research, with significant progress being made in recent years: the in vivo BIA pathway in Escherichia coli and Saccharomyces cerevisiae have been reported with the production of natural BIAs [13] , [14] , [15] , [16] , [17] , [18] . Pathways to BIAs have also been achieved using enzyme cascade reactions in vitro in high yields [19] . The NCS Pictet-Spenglerase reaction is the key step to construct the BIA skeleton in such approaches [13] , [19] . Previous work has established the NCS mechanistic requirement for the arylethylamine meta -hydroxyl group, which binds into the NCS active site, and is deprotonated to enable ring formation [20] , [21] . We have reported a recombinant tyrosinase from Candidatus Nitrosopumilus salaria BD31 ( Cn TYR) able to effectively convert 4 to L-DOPA 5 without the requirement for expensive co-factors, generating the required meta -hydroxyl moeity [19] . Additionally a tyrosine decarboxylase from Enterococcus faecalis DC32 ( Ef TyrDC) was developed for the decarboxylation of 5 and these were used in cascades to generate BIAs (Fig. 1b ). However, such cascades do not have to follow the natural pathway starting from L-tyrosine 4 . They can be designed combining other enzymes in different orders, or other substrates, to enable the production of non-natural BIAs. Here, we show the design of a route to differentially halogenated non-natural BIAs through a parallel cascade and combination strategy, in which arylethylamines and arylacetaldehydes are derived from two different amino acids. To achieve this, a TYR is used to provide the necessary meta -hydroxyl group and a TyrDC to produce the amine from the amino acid. Also, a transaminase (TAm) for aldehyde formation, and finally NCS are used for BIA formation (Fig. 1b ). Importantly, as well as defining the parallel cascade sequence, to extend the enzyme cascades into other substrate capabilities, Cn TYR variants are generated with good monophenolase activities towards halogenated tyrosines, enabling the production of a range of halogenated BIAs. Designing and implementing parallel cascades To generate the required arylethylamine moiety in the upper branch of the parallel cascade (Fig. 2a ), the first step when using L-tyrosine 4 or analogues is the addition of a meta -hydroxyl group. In this one-pot process in initial studies, dopamine 2 was formed in a quantitative yield from 4 . Tyramine 7 could also be formed as an intermediate with both enzymes, if the decarboxylation occurs prior to the hydroxylation. Sodium ascorbate 8 was added to prevent the oxidation of substrates and products, and enzyme lysates were used for ease of production and as these are normally used in industry. Studies confirmed that Ef TyrDC could also be used with meta -L-tyrosine 9 to produce meta -tyramine 10 in >95% yield [19] . Fig. 2: Designing the parallel cascade. a The upper branch to arylethylamines. i. Dopamine 2 was generated in a one-pot two step cascade reaction from L-tyrosine 4 combining Cn TYR and Ef TyrDC; ii. Meta -tyramine 10 was produced from meta -tyrosine 9 by Ef TyrDC; Reaction conditions i: a 1 mL of reaction mixture (50 mM HEPES, pH 5.5) containing 4 (2.5 mM, 1 equiv. ), 0.4 mgmL −1 cell lysate of Cn TYR (containing 21% of recombinant protein), 0.4 mgmL −1 cell lysate of Ef TyrDC (containing 25% of the recombinant protein), sodium ascorbate 8 (4 equiv. ), CuSO 4 (40 μM) and PLP (1.25 mM) at 25 °C, 250 rpm for 6 h and quenched by adding 1 μL of trifluoroacetic acid (TFA). ii: a 1 mL of reaction mixture (50 mM HEPES, pH 7.5) containing 7 (2.5 mM, 1 equiv. ), 0.4 mgmL −1 cell lysate of Ef TyrDC (containing 25% of the recombinant protein), sodium ascorbate 8 (1 equiv.) and PLP (1.25 mM) at 25 °C, 250 rpm for 6 h, and quenched by adding 1 μL of TFA). b The lower branch to the aldehydes. 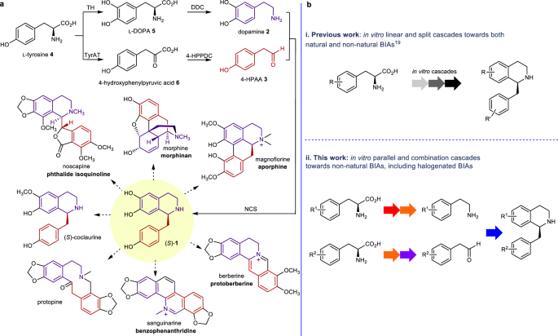Fig. 1: Biosynthetic and biocatalytic routes to BIAs and a parallel cascade adopted in this work. aBiosynthetic BIA pathway in plants and examples of the alkaloid formed. L-Tyrosine4is converted to L-DOPA5by tyrosine hydroxylase (TH), then to dopamine2by DOPA decarboxylase (DDC). In a parallel pathway,4is converted into 4-HPAA3via 4-hydroxyphenylpyruvic acid6by tyrosine aminotransferase (TyrAT) and 4-hydroxyphenylpyruvate decarboxylase (4-HPPDC). Compounds2and3are condensed by the Pictet-Spenglerase norcoclaurine synthase (NCS), generating (S)-norcoclaurine, (S)-1, which is converted into BIAs, such as morphinans, aporphines and protoberberines11,12.bCascade reactions to BIAs inspired by nature: i. Previous work on in vitro assembly of natural and non-natural BIAs from single amino acid substrate. ii. The in vitro parallel cascade to non-natural BIAs reported in this study. See Table 1 for reaction conditions. Full size image For aldehyde production in the lower half of the cascade (Fig. 2b and Table 1 ), readily available starting materials were required, and amino acids were an ideal starting point. Arylacetaldehydes are particularly challenging to prepare as they are oxidatively sensitive and can self-condense via aldol reactions. Here, to produce aldehydes, the transaminase from Chromobacterium violaceum DSM30191 ( Cv TAm) was selected, in combination with Ef TyrDC, as they have both been reported to have broad substrate tolerances [19] , [22] , [23] , [24] . Amino acids 4 , 5 , 9 , 3-F-L-tyrosine 11 , 3-Cl-L-tyrosine 12 and 3-I-L-tyrosine 13 were investigated for aldehyde production and the amine 3-phenyl-1-propylamine 14 was also used. Decarboxylation (other than for 14 ) was followed by deamination with sodium pyruvate 15 as the amine acceptor and pyridoxal 5′-phosphate (PLP) as cofactor. All of the selected substrates were readily accepted by Ef TyrDC and Cv TAm, giving compounds 16 – 22 in overall conversions of 70–95% (Table 1 ). Enzyme lysates were used in all cases. Table 1 Lower branch conversion of amino acids and 14 into aldehydes 16–22 Full size table The final step in this five enzyme-step parallel cascade was combining the amine and aldehyde moieties with addition of a wild-type (WT) Tf NCS enzyme that has displayed good substrate tolerances [25] , [26] . Overall, two amino acids were used as starting materials (other than when utilising 14 ), one for the amine generation (upper branch) and the other for aldehyde formation (lower branch). Nine cascades were constructed, the first five using L-tyrosine 4 (Fig. 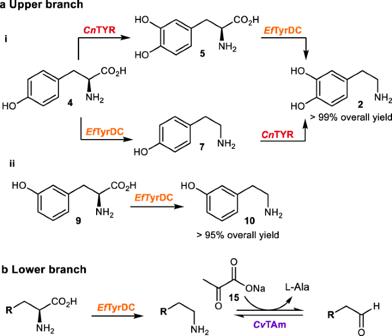Fig. 2: Designing the parallel cascade. aThe upper branch to arylethylamines. i. Dopamine2was generated in a one-pot two step cascade reaction from L-tyrosine4combiningCnTYR andEfTyrDC; ii.Meta-tyramine10was produced frommeta-tyrosine9byEfTyrDC;Reaction conditionsi: a 1 mL of reaction mixture (50 mM HEPES, pH 5.5) containing4(2.5 mM, 1 equiv.), 0.4 mgmL−1cell lysate ofCnTYR (containing 21% of recombinant protein), 0.4 mgmL−1cell lysate ofEfTyrDC (containing 25% of the recombinant protein), sodium ascorbate8(4 equiv.), CuSO4(40 μM) and PLP (1.25 mM) at 25 °C, 250 rpm for 6 h and quenched by adding 1 μL of trifluoroacetic acid (TFA). ii: a 1 mL of reaction mixture (50 mM HEPES, pH 7.5) containing7(2.5 mM, 1 equiv.), 0.4 mgmL−1cell lysate ofEfTyrDC (containing 25% of the recombinant protein), sodium ascorbate8(1 equiv.) and PLP (1.25 mM) at 25 °C, 250 rpm for 6 h, and quenched by adding 1 μL of TFA).bThe lower branch to the aldehydes. See Table1for reaction conditions. 3 , Table 2 , entries 1–5) with Cn TYR and Ef TyrDC for amine production (25 °C, 6 h). In parallel, meta -L-tyrosine 7 (Fig. 3 , Table 2 , entry 1) was used with Ef TyrDC and Cv TAm (37 °C, 6 h), followed by the addition of Tf NCS (37 °C, 8 h). This produced the non-natural BIA ( S )- 23 in 47% isolated yield (82% yield by analytical HPLC) and 90% enantiomeric excess ( ee ). The isolation of BIAs, as reported previously can result in the loss of product, so the conversion yields are also given (determined by HPLC against product standards) [19] , [27] . The cascade to ( S )- 24 [28] was achieved with the aldehyde formed from 14 (Table 2 , entry 2) using Cv TAm, giving ( S )- 24 in 14% isolated yield (21% yield by HPLC) and 90% ee . The lower yield of ( S )- 24 suggested that the wild-type Tf NCS may not accept phenyl propionaldehyde as readily as arylacetaldehydes. Halogenated tyrosines were also adopted into the cascades where 11 , 12 and 13 (Table 2 , entries 3–5) were converted into the corresponding halogenated arylacetaldehydes 19 – 21 , which were then condensed with the amine using Tf NCS, forming halogenated BIAs ( S )- 25 – 27 in 40–42% isolated yield (84–86% yields by analytical HPLC) and up to 96% ee . Fig. 3: Parallel cascades with Cn TYR, Ef TyrDC, Cv TAm, and Tf NCS to non-natural BIAs. The amine moiety was derived from an amino acid (substrate 1) using a Cn TYR- Ef TyrDC cascade. In a parallel pathway, another amino acid (substrate 2) was converted into the aldehyde moiety by a Ef TyrDC- Cv TAm cascade. Non-natural BIAs were then synthesised using Tf NCS. Full size image Table 2 Use of the parallel cascades to produce BIAs 23–31 Full size table In a similar fashion, four parallel cascades starting from meta -L-tyrosine 9 (Table 2 , entries 6–9) to produce the amine moiety were established. In the first of these approaches the starting materials were swapped, compared to entry 1, with L-tyrosine 4 producing the aldehyde 4-HPAA 3 , giving ( S )- 28 in 42% isolated yield (76% yield by HPLC) and 92% ee . Similarly, halogenated L-tyrosines 11 – 13 (Table 2 , entries 7–9) were used to produce the aldehyde and matched with the amine component derived from 9 , giving halogenated BIAs ( S )- 29 – 31 in 27–35% isolated yield (58–68% yield by analytical HPLC). The ee of ( S )- 29 was 85%, slightly lower than for ( S )- 30 (95% ee ) and ( S )- 31 (91% ee ). In general, lower yields for the halogenated BIAs ( S )- 29 – 31 derived from 9 were noted, compared to BIAs ( S )- 25 – 27 generated from 4 , presumably reflecting the more activated dopamine catechol ring that interacts with Lys122 in the NCS active site. Some halogenated BIAs have been reported previously and were produced via a chemoenzymatic route. Maresh et al. [29] utilised the oxidant NaOCl for aldehyde generation to produce 26 and 27 . However, enzymes can react under milder and more environmentally friendly conditions and only relative rates with Tf NCS were described. In addition, in recent work on the synthesis of noscapine in yeast, some C-8 halogenated BIAs were detected by liquid-chromatography mass spectrometry analysis (LC-MS) [30] . Here, the parallel in vitro cascades highlight a versatile amino-acid derived route to halogenated BIA synthesis in high ee s. The tyrosinase ( Cn TYR) used in the enzyme cascades was found to be limiting as L-tyrosine 4 and tyramine 7 were well accepted but 3-F-L-tyrosine 11 was poorly accepted [19] . For wider applications it was desirable to expand the substrate range, however, the iodo-analogue 3-I-L-tyrosine 13 has been reported to be a ‘mixed type’ inhibitor (a competitive and non-competitive inhibitor) for some tyrosinases [31] . 2-Chlorophenol has also been described to act as a competitive inhibitor towards tyrosinases [32] . Therefore, to expand the capability of these cascades using tyrosinases, mutagenesis of Cn TYR was investigated. CnTYR mutagenesis The narrow substrate range of Cn TYR is likely due to steric interactions in the active site, precluding access by the halogenated tyrosines. To probe this, several Cn TYR variants were proposed based on the DNA alignment of Cn TYR with reported engineered tyrosinase variants described by Kanteev et al. [33] (G63L, E185L, N201A, and N201D, Supplementary Fig. 87a ) and Davis et al. [34] , (N132A/L289V, S161I/L163Y, Supplementary Fig. 87b ) respectively. Preliminary global docking studies were initially carried out using AutoDock Vina [35] (Supplementary Methods 10 ), substrates 4 , 9 , and halogenated tyrosines 11 and 12 to investigate the potential of these variants towards halogenated tyrosines. Using the crystal structure of Bm TYR (PDB code: 3NPY) [36] as a template, homology modelling (SWISS-MODEL) [37] was used to develop a model of wild-type Cn TYR. Cn TYR variants were generated in silico using Chimera [38] , [39] , [40] . Residues at 63, 185 and 201 positions of Cn TYR were all located at the entrance of the catalytic site. G63 is already a smaller residue so was not modified (Supplementary Fig. 88a ), while E185 was not modified due to concern of its remote distance to the catalytic site (Supplementary Fig. 87b ). The N201 is a conserved residue in tyrosinases, and is believed to be important for stabilisation of the orientation of the nearby H200 imidazole for Cu coordination; mutation in previous work to Ala or Asp reduced activities. Here, the variant N201S was generated, with the rationale that a switch from the conserved polar residue N to S, might still enable stabilisation of the nearby His residue (Supplementary Fig. 87c ). Residues at N132/L289 and S161/L163 of Cn TYR are located at outer loops (Supplementary Fig. 87d, e ). According to Davis et al. [34] , variant RV145 (equivalent to N132A/L289V) was reported to show a better tolerance towards 4-halophenols and therefore N132A/L289V was also selected for further investigation. The target genes of the two variants were codon optimised for E.coli expression and synthesised (Eurofins TM ). To confirm activities, the Cn TYR variants N132A/L289V and N201S were first screened against the tyrosine analogues, including L-tyrosine 4 , tyramine 7 , meta -L-tyrosine 9 , 3-F-L-tyrosine 11 , 3-Cl-L-tyrosine 12 , 3-I-L-tyrosine 13 , 3-NH 2 -L-tyrosine 32 , 3-NO 2 -L-tyrosine 33 , meta -tyramine 10 , octopamine 34 , synephrine 35 , 4-(2-aminoethyl)aniline 36 , 4-F-L-phenylalanine 37 , 4-Cl-L-phenylalanine 38 , 4-Br-L-phenylalanine 39 , 4-OMe-L-phenylalanine 40 , 4-NH 2 -L-phenylalanine 41 and 4-NO 2 -L-phenylalanine 42 (see Supplementary notes 1 for all structures). A rapid colorimetric screen was used based on the oxidation of 4 and analogues, resulting in the formation of black quinone products (Supplementary Fig. 90a ) [41] . Reactions were performed at 25 °C for 3 h using enzyme lysates and the results indicated (Supplementary Fig. 90b ) that variant N132A/L289V gave no oxidised analogues, suggesting it was inactive. HPLC analysis confirmed that no oxidised products had been formed. Variant N201S, by comparison, showed strong activities towards the natural substrates L-tyrosine 4 and tyramine 7 . Interestingly, the meta -L-tyrosine 9 and 3-Cl-L-tyrosine 12 reactions also turned completely black and with 3-I-L-tyrosine 13 a grey coloration was formed. The substituted phenylalanines 37 – 42 and 33 did not appear to be accepted by either the wild-type Cn TYR or variant N201S. 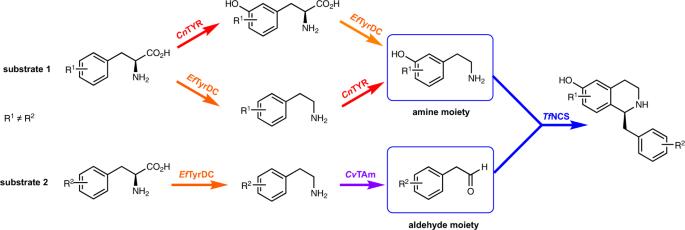Fig. 3: Parallel cascades withCnTYR,EfTyrDC,CvTAm, andTfNCS to non-natural BIAs. The amine moiety was derived from an amino acid (substrate 1) using aCnTYR-EfTyrDC cascade. In a parallel pathway, another amino acid (substrate 2) was converted into the aldehyde moiety by aEfTyrDC-CvTAm cascade. Non-natural BIAs were then synthesised usingTfNCS. Both the wild-type Cn TYR and the variant N201S gave full consumption of L-tyrosine 4 and tyramine 7 , and it was noted that reactions with N201S turned black ~10-times faster than with the wild-type Cn TYR (Table 3 ). The wild-type Cn TYR gave conversions for 3-F-L-tyrosine 11 , 3-NH 2 -L-tyrosine 32 , octopamine 34 , synephrine 35 , and 4-(2-aminoethyl)aniline 36 of 24–51% within 3 h, while the N201S gave >90% conversions with those substrates. Importantly, the wild-type TYR did not accept meta -L-tyrosine 9 , 3-Cl-L-tyrosine 12 , 3-I-L-tyrosine 13 , and meta -tyramine 10 , while the N201S variant gave conversions of 55–64% towards 9 , 12 and 10 and 10% for 13 . Table 3 Comparison of the conversion yields of the wild-type Cn TYR and Cn TYR_N201S towards different substrates Full size table Preliminary molecular docking studies with L-tyrosine 4 and 3-F-L-tyrosine 11 suggested they readily fitted into the active sites of both the wild-type Cn TYR and N201S, with the para -hydroxyl group bound to one of the Cu 2+ ions in the di-copper centre of tyrosinases, allowing the meta -carbon to be hydroxylated by the other Cu 2+ (Fig. 4a, d ). In addition, meta -L-tyrosine 9 and 3-Cl-L-tyrosine 12 could access the enzyme active sites but not in a productive orientation, which agreed with the reported competitive inhibitor behaviour of some substrates with tyrosinases. With the wild-type Cn TYR, 12 was orientated with the para -hydroxyl group and meta -chloro group facing towards to the di-copper centre, with the other meta -carbon faced away from the di-copper centre which can then not be hydroxylated (Fig. 4e ). Similarly, the meta -hydroxyl group of 9 faced away from the di-copper centre in the wild-type Cn TYR (Fig. 4b ). However, with variant N201S, 3-Cl-L-tyrosine 12 was rotated with the meta -chloro group facing away from the di-copper centre, while the para -hydroxyl group and the other meta -carbon faced towards to the catalytic copper. Therefore, here the para -hydroxyl group can bind to one of the coppers and the meta -carbon near to the copper centre can be hydroxylated (Fig. 4f ). Similarly, substrate 9 was orientated with the meta -hydroxyl group facing towards to the Cu 2+ ion, so the nearby ortho -carbon can be hydroxylated (Fig. 4c ) by the variant N201S. Further docking experiments suggested that the smaller size of Ser201 compared to Asn201 may allow the substrates 9 and 12 to be oriented into productive conformations (Supplementary Fig. 89a–c for substrates 9 and 89d-f for substrates 12 ). Fig. 4: Molecular docking studies with WT- Cn TYR and the variant N201S. WT- Cn TYR and the variant N201S (homology modelled) with L-tyrosine 4 , meta -L-tyrosine 9 and halogenated tyrosines 11 and 12 using AutoDock Vina [35] . a Docking of L-tyrosine 4 with the wild-type (WT) Cn TYR and Cn TYR-N201S: L-tyrosine 1 fits well into the active sites of WT- Cn TYR and Cn TYR-N201S. b Docking of meta -L-tyrosine 9 with the WT- Cn TYR: 9 can fit into the active site of WT- Cn TYR but not in a productive orientation. c Docking of 9 with Cn TYR-N201S: 9 fits well into the active site of Cn TYR-N201S. d Docking of 3-F-L-tyrosine 11 with WT- Cn TYR and Cn TYR-N201S: 11 fits well into the active site of both. e Docking of 3-Cl-L-tyrosine 12 with WT- Cn TYR: 12 can fit into the active sites WT- Cn TYR but not in a productive orientation. f Docking of 12 with Cn TYR-N201S: 12 fits well into the active sites of Cn TYR-N201S. The functional histamine residues in the tyrosinase active sites and substrates are shown in stick and ribbon forms. Enzyme residues are shown in tan. Compounds 4 , 9 , 11 , and 12 are shown in grey, rose, blue, and light blue, respectively. The model of WT- Cn TYR was generated by homology modelling (SWISS-MODEL) [37] using the crystal structure of Bm TYR (PDB code: 3NPY) [36] as a template. Cn TYR variants were generated and homology modelled by Chimera [38] , [39] , [40] . Full size image Kinetic studies with Cn TYR-N201S revealed the apparent kinetic parameters K m, app . and k cat,app . towards L-tyrosine 4 were 1.89 mM and 182.9 s −1 ( k cat,app ./ K m, app . 9.68 × 10 4 s −1 M −1 ) and the corresponding values for tyramine 7 were 1.78 mM and 197.5 s −1 ( k cat,app. / K m, app . 1.11 × 10 5 s −1 M −1 ), respectively. Compared to the wild-type Cn TYR ( k cat,app ./ K m,app . 1.78 × 10 4 s −1 M −1 towards 4 and 1.61 × 10 4 s −1 M −1 towards 7 ) [19] , the catalytic efficiencies of Cn TYR-N201S towards both 4 and 7 were 6-fold higher. This could be due to the larger size of the entrance into the active site, enhancing access for substrates 4 and 7 , but would also make it easier for the catechol substrates to access the active site, boosting the diphenolase reaction and over-oxidation of catechols to quinones. While the highest yield of L-DOPA 5 produced by the variant with 4 was 76% (using optimised conditions), 10 equivalents of sodium ascorbate 8 were required. The large amounts of ascorbate added could cause problems during product purifications so the generation of new variants maintaining a higher monophenolase activity was explored. Directed evolution based on Cn TYR-N201S were then carried out for this purpose. Random mutagenesis was performed with E. coli XL 1-Red cells and twenty-six stable and positive colonies resulted after three rounds of re-transformation and colorimetric selection (see the methods section). Compounds 3-F-L-tyrosine 11 and 3-Cl-L-tyrosine 12 were screened with sodium ascorbate 8 under different concentrations (0, 4, and 10 equiv.) and used to select appropriate variants. The enzyme monophenolase activities were initially estimated based on the colorimetric assay: if the reaction turned black without 8 and slightly brown with 4 equiv. of 8 , this suggested potentially a better monophenolase activity towards the substrate. All negative controls gave rise to no colour change. Variants M1 and M23–M25 were estimated to display a better monophenolase activity towards 11 , while M8 and M26 gave higher monophenolase activities towards 3-Cl-L-tyrosine 12 (Fig. 5a ). Fig. 5: Directed evolution based on CnTYR-N201S and enzyme screening data. a Enzyme screening for the random mutagenized variants based on Cn TYR-N201S with 3-F-L-tyrosine 11 and 3-Cl-L-tyrosine 12 . Reaction conditions : 11 and 12 (2.5 mM, 1 equiv. ), enzyme lysates (400 μgmL −1 ) and CuSO 4 (5 μM) with 0, 4 equivalents and 10 equivalents of sodium ascorbate 8 , respectively. Reactions were performed at 25 °C for 8 h. The black colour indicates the diphenolase activities of the tyrosinases. Note: WT- Rs TYR ( Rs ) [19] , Cn TYR ( Cn ), and Cn TYR-N201S (N201S) lysates were used as positive controls and cell lysates of an empty plasmid as a negative control (NC). b Product yields and components of TYR reactions with 4 equiv. of 8 using WT- Cn TYR and Cn TYR variants towards 3-F-L-tyrosine 11 : orange bars represent the catechol product 3-F-L-DOPA 43 by HPLC against product standards, and the blue bars represent the over-oxidation products (determined by analytical HPLC with short retention times). c Product yields and components of TYR reactions with 4 equiv. of 8 using WT- Cn TYR and Cn TYR variants towards 3-Cl-L-tyrosine 12 : pink bars represent the catechol product 3-Cl-L-DOPA 44 by HPLC against product standards, and the grey bars represent the over-oxidation products as determined by analytical HPLC. Experiments were performed in triplicates. Error bars indicate the standard error of the triplicate reactions. Full size image The quantification of products generated by the selected variants with 4 equiv. of ascorbate 8 was then carried out. Variant M1 gave the highest yield of the catechol product 3-F-L-DOPA 43 , with a 90% yield by HPLC analysis (Fig. 5b ), followed by variant M25 and wild-type Cn TYR (70% yield). Variants M8 and M26 gave the highest amount of 3-Cl-L-DOPA 44 in 55–60% yield (Fig. 5c ). Variants M1, M8, M25, and M26 were sequenced as N201S/G205R/V206I, N201S/H202N, N201S/G205R and N201S/G205K, respectively. This indicated that on changing Gly205 to residues, Arg or Lys, the diphenolase activities were decreased, possibly due to steric reasons, with these groups obstructing the catechol products from re-entering the active sites. A similar effect was also observed in a previous study on the mutagenesis of Bm TYR: when they mutated the residues Met61, Met184, and Phe197, which are located at the entrance to the active site, to the smaller residues Leu and Ala (M61L, M184L, and F197A), the diphenolase activity was enhanced [33] . Electrostatic interactions may also be important. It has been reported that the Asn201 residue is highly conserved among tyrosinases, however, its role is still unclear [33] , [34] , [42] . According to Kanteev et al. [33] , the Asn residue may stabilise the nearby His residue and coordinate with Cu 2+ for its uptake, and the substitution of this to either Ala or Asp decreased Bm TYR activities. However, the substitution of Asn201 to Ser in Cn TYR increased the enzyme activities in this study. This could possibly be due to the Ser201 forming a hydrogen bond with the imidazole ring of the nearby His200 residue, orientating the His residue into a position for better Cu 2+ uptake. Meanwhile, the smaller size of the Ser201 can allow bulkier substrates to access the active site. Although N201S is a successful candidate for the acceptance of 3-F-L-tyrosine 11 and 3-Cl-L-tyrosine 12 , preliminary docking analysis was insufficient to reveal the function of Ser201. In the future, further experiments using MD simulation studies may provide further insights. The variants generated were then used in the BIA cascades. Use of CnTYR variants in BIA synthesis Initially the TYR were tested in cascades based upon those previously established, providing ( S )- 45 (in 35% HPLC yield) [19] and ( S )- 46 (in 27% HPLC yield) [43] from 11 using wild-type Cn TYR, Ef TyrDC, phenylacetaldehyde 47 and Tf NCS, and for ( S )- 46 a methyltransferase (MT). The tyrosinase reaction previously limited the yields in these enzyme cascades. Notably, when replacing wild-type Cn TYR with the variants N201S, M1(N201S/G205R/V206I), and M25 (N201S/G205R), the yield of ( S )- 45 increased to 66, 89, and 79% by HPLC analysis, respectively (Fig. 6a ). The highest yield reached was 89% with the variant N201S/G205R/V206I. Meanwhile, the yield of ( S )- 46 reached 77–86% (by HPLC analysis) using Cn TYR-M1 (N201S/G205R/V206I) (Fig. 6b ). For the final methylation step, three O -MTs were trialled, the catechol- O -MTs from Rattus norvegicus ( Rn COMT) [44] and Coptis japonica ( Cj -6-OMT) [45] , [46] , and SafC from Myxococcus xanthus ( Mx SafC) [47] with all giving the 6-OMe product 46 in good yields [43] . Due to the high cost of the cofactor ( S )-adenosylmethionine (SAM), a methionine adenosyltransferase (MAT E.C. 2.5.1.6) was used to generate SAM from ATP and L-methionine, and a methylthioadenosine nucleosidase (MTAN, E.C. 3.2.2.9.) to remove the inhibitory by-product ( S )-adenosylhomocysteine (SAH), both from E. coli ( Ec ) [48] . Reaction times for the tyrosinase steps were also shortened to 8 h compared to 24 h using the wild-type enzyme. A similar three enzyme cascade was then established starting from 3-Cl-L-tyrosine 12 . The Cn TYR variants N201S, M8 (N201S/H202N) and M26 (N201S/G205K) were investigated in the cascade and gave the chlorinated alkaloid ( S )- 48 in 35–45% yield (Fig. 6c ). Variant N201S/H202N gave the highest yield for ( S )- 48 of 45% (by HPLC analysis) and 92% ee . Interestingly, when using meta -L-tyrosine 9 as the starting material in this three-enzyme cascade comprising Cn TYR-N201S, Ef TyrDC and Tf NCS, 49 was generated, indicating that Cn TYR-N201S hydroxylated the ortho - and more sterically hindered carbon of 9 (Fig. 6d ), to give a non-natural alkaloid. Fig. 6: Production of alkaloids ( S )-45,46,48 and 49 using Cn TYR variants. a Production of ( S )- 45 using WT- Cn TYR, variants N201S, M1 (N201S/G205R/V206I) and M25 (N201S/G205R). b Production of ( S )- 46 using WT- Cn TYR and M1 (N201S/G205R/V206I) together with MTs Rn COMT/ Mx SafC/ Cj 6OMT, Ec MAT (SAM supply), and Ec MTAN (SAH degradation). c Production of ( S )- 47 using WT- Cn TYR, N201S, M8 (N201S/H202N) and M26 (N201S/G205K). d Production of ( S )- 48 using WT- Cn TYR, N201S, M1 (N201S/G205R/V206I) and M8 (N201S/H202N). e Enzyme cascades to alkaloids ( S )− 45 , 46 , 48 , and 49 . Reaction conditions : Details are provided in the Supplementary Information and are specific to each cascade. E.g., for ( S )- 46 , a 20 mL reaction mixture of 11 (10 mM, 1 equiv. ), Cn TYR variants and Ef TyrDC lysates (10% (v/v)), 8 (4 equiv.) PLP (5 mM) and CuSO 4 (5 μM) at 25 °C for 8 h. Compound 47 (1.5 equiv.) and Tf NCS lysates (10% (v/v)) were then added for another 16 h reaction. For the methylation step, Ec MAT lysates (10% (v/v)), Ec MTAN lysates (2.5% (v/v)) and Rn COMT/ Mx SafC/ Cj 6OMT lysates (10% (v/v)) were added for another 8 h reaction. a Yields were determined by HPLC analysis at 280 nm against products standards. Experiments were performed in triplicate, and the error bars indicate the standard error of the triplicate reactions; b Isolated yields are given in parenthesis for preparative-scale reactions and products were purified by preparative HPLC or an extraction method; c ee s were determined by chiral HPLC. Full size image Meanwhile, to determine whether the yields of the halogenated alkaloids could be enhanced further, the Tf NCS variants, L76V, A79I, A79F, F80L, M97F, and A182I, were also investigated in the three-enzyme cascades to give 45 and 48 (Fig. 6e ). The variant A79I gave the halogenated alkaloids ( S )- 45 and ( S )- 48 in slightly higher yields than the wild-type Tf NCS, in 92 and 48% yields by HPLC analysis, respectively (see SI, S12) whereas the others were similar or lower [26] , [49] , [50] . Preliminary docking studies were also performed with the wild-type and A79I- Tf NCS which suggested that the variant A79I folds the iminium carbon in closer proximity to the carbon ortho - to the F/Cl on the aromatic ring of halogenated BIA intermediates, which could account for this observation (see Supplementary Table 2 , 3.90 Å for ( S )- 45 )/3.78 Å (for ( S )- 46 with A79I, and 4.77 Å for ( S )- 45 )/4.68 Å for ( S )- 46 with the wild-type). The enzyme cascades were then extended using halogenated tyrosines as the starting materials, and for the production of aldehydes. Arylethylamines were generated from 11 and 12 as before using Cn TYR-M1 (N201S/G205R/V206I) and Cn TYR-M8 (N201S/H202N), respectively, and Ef TyrDC. Arylacetaldehydes were derived from Ef TyrDC and Cv TAm, and when synthesised Tf NCS-A79I was used for catalysing the Pictet-Spengler reactions due to the slightly higher yields noted above. 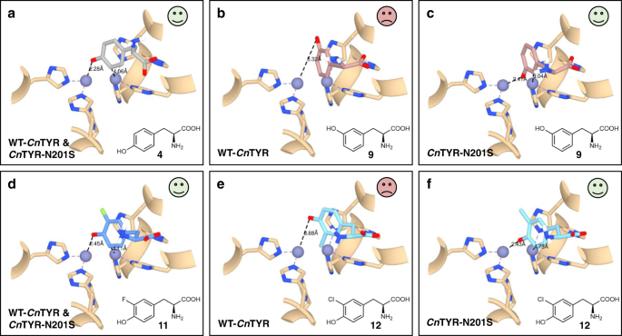Fig. 4: Molecular docking studies with WT-CnTYR and the variant N201S. WT-CnTYR and the variant N201S (homology modelled) with L-tyrosine4,meta-L-tyrosine9and halogenated tyrosines11and 12 using AutoDock Vina35.aDocking of L-tyrosine4with the wild-type (WT)CnTYR andCnTYR-N201S: L-tyrosine1fits well into the active sites of WT-CnTYR andCnTYR-N201S.bDocking ofmeta-L-tyrosine9with the WT-CnTYR:9can fit into the active site of WT-CnTYR but not in a productive orientation.cDocking of9withCnTYR-N201S:9fits well into the active site ofCnTYR-N201S.dDocking of 3-F-L-tyrosine11with WT-CnTYR andCnTYR-N201S:11fits well into the active site of both.eDocking of 3-Cl-L-tyrosine12with WT-CnTYR:12can fit into the active sites WT-CnTYR but not in a productive orientation.fDocking of12withCnTYR-N201S:12fits well into the active sites ofCnTYR-N201S. The functional histamine residues in the tyrosinase active sites and substrates are shown in stick and ribbon forms. Enzyme residues are shown in tan. Compounds4,9,11, and12are shown in grey, rose, blue, and light blue, respectively. The model of WT-CnTYR was generated by homology modelling (SWISS-MODEL)37using the crystal structure ofBmTYR (PDB code: 3NPY)36as a template.CnTYR variants were generated and homology modelled by Chimera38,39,40. Initially 11 and 12 were reacted with 2-bromo-phenylacetaldehyde 50 , giving double halogenated BIAs ( S )- 51 and ( S )- 52 in 83 and 16% yield by HPLC and >92% ee , respectively (Table 4 , entries 1 and 2). The low yield of ( S )- 52 was most likely due to the lower monophenolase activity of the Cn TYR variant with 12 and the effect of the more sterically hindered 3-Cl-dopamine derived intermediates in the NCS active site. More halogenated BIAs were then produced using the ‘parallel cascade’ strategy. The amine moiety was generated from 11 as before, and aldehydes produced from 11 to 13 and 4 (Table 4 , entries 3–7). This gave BIAs ( S )- 54 – 57 in 26–78% yields and >90% ee . Although some of the products were formed in lower yields due to the difficulties of using more sterically challenging halogenated analogues and unknown side-products, it nevertheless highlights a very valuable and flexible strategy to non-natural BIAs in high enantioselectivities. Table 4 Parallel cascades with Cn TYR variants, Ef TyrDC, Cv TAm, and Tf NCS-A79I to halogenated BIAs Full size table In summary, Ef TyrDC and Cv TAm are capable of accepting a broad range of aromatic amino acids, and so were used here to generate aldehydes for coupling reactions using Pictet-Spenglerases. Such arylacetaldehydes are difficult to synthesise using traditional chemical routes as the aldehydes are prone to oxidations and aldol self-condensations. Enzyme cascades were then developed using parallel reaction strategies and nine non-natural BIAs were initially produced in good yields and ee s. Mutagenesis studies were then applied with Cn TYR to expand its substrate scope towards halogenated amino-acids. Several Cn TYR variants were generated that displayed better monophenolase activities towards 3-F-L-tyrosine 11 and accepted meta -L-tyrosine 9 and 3-Cl-L-tyrosine 12 , which are known inhibitors for wild-type tyrosinases. Then extended enzyme cascades using the Cn TYR and Tf NCS variants were carried out to give 14 halogenated (and 13 non-natural) BIAs in good stereoselectivities. Importantly, this is the first time that double halogenated BIAs have been reported, highlighting the abilities of enzyme cascades to ‘mix and match’ arylethylamines and aldehydes to give different BIAs. This parallel enzyme cascade strategy together with enzyme mutagenesis is a powerful synthetic approach for alkaloid synthesis. Chemicals Dopamine 2 , L-tyrosine 4 , L-DOPA 5 , tyramine 7 , sodium ascorbate 8 , 3-Cl-L-tyrosine 12 , 3-I-L-tyrosine 13 , 3-phenyl-1-propylamine 14 , sodium pyruvate 15 , 3-NH 2 -L-tyrosine 32 , 3-NO 2 -L-tyrosine 33 , octopamine 34 , synephrine 35 , 4-(2-aminoethyl)aniline 36 , 4-F-L-phenylalanine 37 , 4-Cl-L-phenylalanine 38 , 4-Br-L-phenylalanine 39 , 4-OMe-L-phenylalanine 40 , 4-NH 2 -L-phenylalanine 41 , 4-NO 2 -L-phenylalanine 42 , PLP, CuSO 4 · 5H 2 O and kanamycin were purchased from Sigma-Aldrich (Germany). Meta -L-tyrosine 9 , meta -tyramine 10 , 3-F-L-tyrosine 11 , phenylacetaldehyde 47 , 2-bromophenylacetaldyhyde 50 and IPTG was purchased from Alfa Aesar (Thermo Fisher Scientific, USA). All chemicals were purchased in the highest purity available. Thin layer chromatography was performed using plates with a silica gel matrix on an aluminium support. Ultraviolet light (254 nm) and ninhydrin stain was used to visualise the plates. HPLC methods Analytical methods were performed with a Dionex TM UltiMate TM 3000 HPLC System, with a Dionex TM UltiMate TM 3000 RS Pump, a Dionex TM UltiMate TM 3000 Autosampler, a Dionex TM UltiMateTM 3000 Column Compartment and a UltiMate TM 3000 RS Diode Array Detector (Thermofisher Scientific, US). Preparative methods were developed with a Agilent 1260 Infinity TM HPLC System, with a 1260 Infinity TM Preparative Pump, a 1260 Infinity TM Preparative-scale Fraction Collector, a 1260 Infinity TM Multiple Wavelength Detector, and a 1260 Infinity TM Preparative Autosampler. Analytical HPLC method 1 (achiral) Achiral quantitative analyses adopted a reverse phase analysis method. Separation was achieved with an ACE 5 C18 column (150 × 4.6 mm) with a flow speed of 1 mL/min at 30 °C. The injection volume was 10 μL. Substrates and products were measured via UV absorbance at 280 nm. Eluent A (H 2 O with (v/v) 0.1% TFA) and eluent B (acetonitrile) were used as a mobile phase over 10 min. The gradient was as: 0.0 min (10% B)-1.0 min (10% B)-6.0 min (70 % B)-6.1 min (100% B)-6.5 min (100% B)-6.6 min (10% B)-10.0 min (10% B). Analytical HPLC method 2 (chiral) The chiral separation was achieved with an Supelco Astec Chirobiotic TM T column (25 cm × 4.6 mm) or a Supelco Astec Chirobiotic TM T2 column (25 cm × 4.6 mm), and a flow speed of 1 mL/min at 30 °C. The injection volume was 5 μL. Products were measured via UV absorbance at 230 nm. Methanol (0.2% AcOH, 0.1% TEA) was used as a mobile phase over 40 min or 80 min. Analytical HPLC method 3 (chiral) The chiral separation was achieved with a Supelco Astec Chirobiotic TM T column (25 cm × 4.6 mm) and a flow speed of 0.2 mL/min at 30 °C. The injection volumes were 5 µL. Compounds were detected by UV absorbance at 230 nm. An isocratic mobile phase 20 mM NH 4 OAc (pH 4.0):MeOH (70:30) was used over 120 min. Preparative HPLC method 4 The separation was achieved with a Vydac TM 218TP1022 (C18, 10 µm, 2.2 cm ID × 25 cm L) preparative column or a Supelco TM Discovery BIO wide pore (C18, 10 µm, 2.12 cm × 25 cm) preparative column and a flow speed of 8 mL/min at 25 °C. The injection volume was 900 μL. Products were identified via UV absorbances at 214 nm and 280 nm. Eluent A (H 2 O with 0.1% (v/v) TFA) and eluent B (acetonitrile with 0.1% (v/v) TFA) were used as a mobile phase over 28 min. The gradient was as: 0.0 min (5 % B)-3.0 min (5% B)-20.0 min (70% B)-22.0 min (70% B)-23.0 min (5% B)-28.0 min (5% B). Preparative HPLC method 5 The separation was achieved with a VydacTM 218TP1022 (C18, 10 µm, 2.2 cm ID × 25 cm L) preparative column or a SupelcoTM Discovery BIO wide pore (C18, 10 µm, 2.12 cm × 25 cm) preparative column and a flow speed of 8 mL/min at 25 °C. The injection volume was 900 μL. Products were identified via UV absorbances at 214 and 280 nm. Eluent A (H 2 O with 0.1% (v/v) TFA) and eluent B (acetonitrile with 0.1% (v/v) TFA) were used as a mobile phase over 28 min. The gradient was as: 0.0 min (25% B)-3.0 min (25% B)-20.0 min (90% B)-22.0 min (90% B)-23.0 min (25% B)-28.0 min (25% B). Chemical analytics 1 H and 13 C NMR spectra were obtained using a Bruker Advance III 700 MHz spectrometer. Chemical shifts specified are relative to trimethylsilane (set at 0 ppm) and referenced to the residual, protonated NMR solvent. Coupling constants in 1 H-NMR spectra ( J ) are given in Hertz (Hz) and described as singlet (s), doublet (d), doublet of doublets (dd), triplet (t), quartet (q), multiplet (m). Mass spectrometry data of compounds were measured on an Agilent 1100 Series System with a Finnigan LTQ mass spectrometer. An ACE 5 C18 reverse phase column (50 mm × 2.1 mm, 5 μm) was adopted with a mobile phase of eluent A (H 2 O with 0.1% (v/v) formic acid) and eluent B (acetonitrile) over 5 min with a flow rate of 0.6 mL/min. The sample injection volume was 10 μL. Chemical compounds were measured in a positive ion mode, and the operating conditions of the ESI interface were set to a capillary temperature 300 °C, capillary voltage 9 V, spray voltage 4 kV, sheath gas 40, auxiliary gas 10, sweep gas 0 arbitrary units. The gradient of eluents was as: 0.0 min (5% B)-4.0 min (90% B)-4.5 min (5% B)-5.0 min (5% B). Recombinant protein expression in E. coli BL21 (DE3) Selected enzyme glycerol stocks ( E. coli BL21 (DE3)) were plated out on agar plates supplemented with 50 µg/mL kanamycin. A single colony was then picked to inoculate into 10 mL of LB media supplemented with 50 µg/mL kanamycin and grown at 37 °C and 250 rpm overnight (8–16 h). 1 mL of the overnight cultures were inoculated into a 500 mL baffled shaking flask containing 100 mL of TB media supplemented with 50 μg/mL kanamycin at 37 °C, 250 rpm until an OD 600 = 0.6. Enzyme expression was induced by the addition of 1 mM IPTG (and 100 μM CuSO 4 · 5H 2 O for Cn TYR) to the culture. Cultures were incubated overnight at 25 °C prior for harvesting, whilst shaking at 250 rpm. Cells were harvested by centrifugation (12,000 × g , 15 min) and the cell pellets was stored at −20 °C Cell lysate preparation Cell pellets (50 mL culture) were resuspended in 5 mL of 50 mM HEPES buffer (pH 5.5/pH7.5) and lysed by 10 cycles of sonication on ice (10 s on plus 10 s off, 12 watts output) equipped with a Process Timer. Cell lysates were then centrifuged at 4 °C (12,000 × g , 15 min). The supernatant was collected and buffer exchanged using SephadexTM G-25 in PD-10 column (GE Healthcare Life Sciences, Germany) with HEPES buffer (50 mM, pH 5.5/pH7.5) to remove the KPi in cell components. The concentration of supernatant protein was measured following the standard Bradford procedure. The samples were duplicated and the average OD 595 were used for cell lysate concentration calculations. 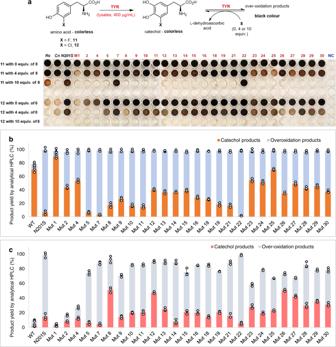Fig. 5: Directed evolution based on CnTYR-N201S and enzyme screening data. aEnzyme screening for the random mutagenized variants based onCnTYR-N201S with 3-F-L-tyrosine11and 3-Cl-L-tyrosine12.Reaction conditions:11and12(2.5 mM, 1 equiv.), enzyme lysates (400 μgmL−1) and CuSO4(5 μM) with 0, 4 equivalents and 10 equivalents of sodium ascorbate8, respectively. Reactions were performed at 25 °C for 8 h. The black colour indicates the diphenolase activities of the tyrosinases. Note: WT-RsTYR (Rs)19,CnTYR (Cn), andCnTYR-N201S (N201S) lysates were used as positive controls and cell lysates of an empty plasmid as a negative control (NC).bProduct yields and components of TYR reactions with 4 equiv. of8using WT-CnTYR andCnTYR variants towards 3-F-L-tyrosine11: orange bars represent the catechol product 3-F-L-DOPA43by HPLC against product standards, and the blue bars represent the over-oxidation products (determined by analytical HPLC with short retention times).cProduct yields and components of TYR reactions with 4 equiv. of8using WT-CnTYR andCnTYR variants towards 3-Cl-L-tyrosine12: pink bars represent the catechol product 3-Cl-L-DOPA44by HPLC against product standards, and the grey bars represent the over-oxidation products as determined by analytical HPLC. Experiments were performed in triplicates. Error bars indicate the standard error of the triplicate reactions. 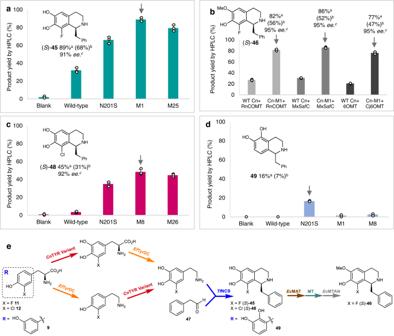Fig. 6: Production of alkaloids (S)-45,46,48 and 49 usingCnTYR variants. aProduction of (S)-45using WT-CnTYR, variants N201S, M1 (N201S/G205R/V206I) and M25 (N201S/G205R).bProduction of (S)-46using WT-CnTYR and M1 (N201S/G205R/V206I) together with MTsRnCOMT/MxSafC/Cj6OMT,EcMAT (SAM supply), andEcMTAN (SAH degradation).cProduction of (S)-47using WT-CnTYR, N201S, M8 (N201S/H202N) and M26 (N201S/G205K).dProduction of (S)-48using WT-CnTYR, N201S, M1 (N201S/G205R/V206I) and M8 (N201S/H202N).eEnzyme cascades to alkaloids (S)−45,46,48, and49.Reaction conditions: Details are provided in theSupplementary Informationand are specific to each cascade. E.g., for (S)-46, a 20 mL reaction mixture of11(10 mM, 1 equiv.),CnTYR variants andEfTyrDC lysates (10% (v/v)),8(4 equiv.) PLP (5 mM) and CuSO4(5 μM) at 25 °C for 8 h. Compound47(1.5 equiv.) andTfNCS lysates (10% (v/v)) were then added for another 16 h reaction. For the methylation step,EcMAT lysates (10% (v/v)),EcMTAN lysates (2.5% (v/v)) andRnCOMT/MxSafC/Cj6OMT lysates (10% (v/v)) were added for another 8 h reaction.aYields were determined by HPLC analysis at 280 nm against products standards. Experiments were performed in triplicate, and the error bars indicate the standard error of the triplicate reactions;bIsolated yields are given in parenthesis for preparative-scale reactions and products were purified by preparative HPLC or an extraction method;cees were determined by chiral HPLC. Determination of target protein concentrations in cell lysates The recombinant proteins were expressed and analysed by SDS-PAGE. Then the SDS gel was analysed with a AlphaImagerTM gel documentation system (ProteinSimple, US), and the recombinant protein concentration present in the cell lysate was determined by AlphaView TM FluorChem Q TM software (ProteinSimple, US). Mutagenesis methods Site-direct mutagenesis of CnTYR Protein and DNA Alignment of the Cn TYR used in this study and the reported TYR was performed with the online service ‘Clustal Omega’ from EMBL-EBI (Cambridgeshire, UK). Alignment results were shown using the online service ‘Sequence Manipulation Suite’ from the University of Alberta (Alberta, CA). Genes for the designed mutants were synthesised from Eurofins Scientific (Belgium). Random mutagenesis of CnTYR Random mutagenesis was performed with E. coli XL 1-Red competent cells purchased from Agilent Technologies TM (Santa Clara, US). Mutation procedures followed the instruction manual. After mutation, plasmids were extracted using the Qiagen Mini Prep KitTM (Qiagen, Germany) and further transformed with E. coli BL21 (DE3) competent cells. After cultivation at 37 °C for 1 h, cells were plated on the LB agar plate with 50 μg/mL kanamycin and 500 μM IPTG. The plates were cultivated at 37 °C overnight. Colonies shown black colour were selected and inoculated in 10 mL of TB broth with 50 μg/mL kanamycin at 37 °C overnight. As a single colony may contain various plasmids, to obtain the stable mutants, again, plasmids were extracted and transformed with E. coli BL21 (DE3) competent cells, which was then plated on the LB agar plates with 50 μg/mL kanamycin and 500 μM IPTG and grown overnight. The above steps were repeated twice. Afterwards, colonies shown black were chosen and further cultivated in TB broth. Mutated proteins were expressed, and cell lysates were used for enzyme screening with 3-F-L-tyrosine 11 and 3-Cl-L-tyrosine 12 based on the colorimetric reaction. The DNA of the selected mutants were sequenced by ‘DNA Sequencing Service’ from Eurofins Scientific (Belgium). Reporting summary Further information on research design is available in the Nature Research Reporting Summary linked to this article.